Flexible concentrator photovoltaics based on microscale silicon solar cells embedded in luminescent waveguides Unconventional methods to exploit monocrystalline silicon and other established materials in photovoltaic (PV) systems can create new engineering opportunities, device capabilities and cost structures. Here we show a type of composite luminescent concentrator PV system that embeds large scale, interconnected arrays of microscale silicon solar cells in thin matrix layers doped with luminophores. Photons that strike cells directly generate power in the usual manner; those incident on the matrix launch wavelength-downconverted photons that reflect and waveguide into the sides and bottom surfaces of the cells to increase further their power output, by more than 300% in examples reported here. Unlike conventional luminescent photovoltaics, this unusual design can be implemented in ultrathin, mechanically bendable formats. Detailed studies of design considerations and fabrication aspects for such devices, using both experimental and computational approaches, provide quantitative descriptions of the underlying materials science and optics. Optical concentration represents a strategy for collecting incident solar radiation and redirecting it onto photovoltaic (PV) cells to increase their output power [1] , [2] . These techniques are of interest because they can reduce costs by improving the utilization of the cells and, in certain cases, by raising their efficiencies [3] . Conventional concentrators use focusing lenses and mechanical devices (that is, trackers) to maintain alignment with incident solar radiation [4] , [5] . This design can be attractive, particularly, when implemented with high efficiency compound semiconductor PV cells. Disadvantages, compared with non-concentrating PV, arise from complexity associated with the optics and trackers, challenges in module assembly, difficulties in thermal management and inefficiencies in the capture of diffuse light. Recently developed microscale compound semiconductor multijunction cells, miniaturized optics and advanced manufacturing approaches address many of these issues [6] . Even these systems do not, however, function effectively in geographic locations where levels of direct normal irradiance are low, or in applications that demand mechanically flexible modules. Luminescent solar concentrators (LSCs), by contrast, exploit different optical mechanisms, with the potential to avoid these limitations [7] , [8] , [9] . A simple LSC consists of a planar, multimode slab waveguide doped with a luminescent species. These dopants, referred to as luminophores, absorb incident light and then re-emit at longer wavelengths, in a process of optical down-conversion. The emitted photons have an isotropic angular distribution; those that satisfy the condition of total internal reflection (TIR) at the boundaries of the LSC slab are trapped in guided modes of the structure. Photons that do not meet this TIR condition can be also captured, though less effectively, by coupling into leaky modes [10] , [11] . In a typical arrangement, strips of solar cells mount on the edges of an LSC structure to collect emergent radiation. Although relatively inefficient with direct normal irradiance, this process offers levels of concentration that exceed those possible based on focusing of diffuse light, even in the thermodynamic limit [12] . Also, trackers are not required, thereby reducing the complexity and cost, and creating the possibility for mechanically flexible module designs. Despite these advantages, LSCs have many drawbacks; prominent among these are optical inefficiencies that stem from re-absorption of light emitted by the luminophores and from propagation losses due to scattering and leaky waveguiding [13] . The first effect results from partial overlap of the absorption and emission spectra of the luminophore. This overlap can be reduced with materials (for example, semiconductor quantum dots) [14] , [15] that have large Stokes shifts, or with alternative conversion processes based on near-field energy transfer [16] or phosphorescence [17] . The waveguide losses can be decreased by increasing the difference between the index of refraction of the LSC material and its surroundings, and by engineering the structures to avoid scattering. Pursuing these and other directions represent activities in ongoing research. An important feature of these sources of loss is that their effects diminish with propagation distance. In conventional devices, the cells and the LSC waveguides are bulk components, such that reducing critical dimensions to scales less than several centimeters is impractical. As a result, the geometries of key components in the system cannot be fully exploited as design parameters for optimizing the behaviour. Another restriction of existing structures is that they cannot be implemented effectively with LSC thicknesses in the range required (~200 μm or less) for mechanically flexible construction, due to practical difficulties in mounting cells on narrow edges and to increased levels of self-absorption that result from high luminophore concentrations needed to achieve sufficient optical density in thin layers. Here we present an approach that overcomes both classes of constraints, through the use of a composite material structure consisting of sparse, distributed arrays of microscale solar cells (μ-cells) embedded directly into the LSC waveguide. A key feature is that the dimensions and designs of the μ-cells allow capture of light not only through their top surfaces, but also through their sidewalls and bottom surfaces. Deterministic assembly techniques offer practical access to spacings and array configurations that can match the intrinsic loss characteristics of nearly any type of LSC, even those with extremely small thicknesses (for example, 10 μm or larger), for low-bending stiffness and high degrees of flexibility. 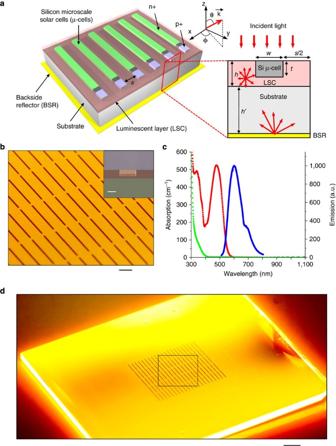Figure 1: A luminescent concentrator system with an array of surface-embedded monocrystalline silicon solar μ-cells. (a) Schematic illustration of a device, consisting of an array of solar microcells (μ-cells), a luminescent layer (LSC layer), a supporting, transparent substrate and a BSR. The inset on the right shows a cross sectional view, with key parameters identified, including width (w) and thickness (t) of the μ-cells, distance (s) between them, thickness (h) of the LSC layer, and thickness (h′) of the substrate. (b) Magnified optical image of arrays of μ-cells printed into a photocured layer of polyurethane (PU) doped with the luminophore DCM, (scale bar: 500 μm). Inset, cross-sectional s.e.m. image (coloured) showing substrate (green), DCM-PU (red), Si μ-cell (yellow), and air (blue), (scale bar: 25 μm). (c) Absorption and emission spectra of a DCM-PU thin film (thickness ~30 μm) on a glass substrate (thickness ~1 mm), with a DCM concentration of ~0.19 wt% (red: absorption of DCM-PU, green: absorption of PU, blue: emission of DCM-PU). (d) Picture of a completed module, before forming interconnects. The dashed box in the centre corresponds to the region shown in frame (b), the scale bar in this image is 2 mm. Luminescent solar concentrator with surface-embedded silicon solar μ-cells Figure 1a shows features of a representative system. The module consists of an array of monocrystalline, ultrathin (10–20 μm) silicon μ-cells, conformally integrated at the surface of a thin layer doped with luminophores and coated on a transparent substrate with a scattering/reflecting element placed on its back surface. Key dimensional parameters include the thickness ( t ) and width ( w ) of the μ-cells, the separation ( s ) between them and the thickness of the luminescent layer ( h ) and substrate ( h ′). Figure 1: A luminescent concentrator system with an array of surface-embedded monocrystalline silicon solar μ-cells. ( a ) Schematic illustration of a device, consisting of an array of solar microcells (μ-cells), a luminescent layer (LSC layer), a supporting, transparent substrate and a BSR. The inset on the right shows a cross sectional view, with key parameters identified, including width ( w ) and thickness ( t ) of the μ-cells, distance ( s ) between them, thickness ( h ) of the LSC layer, and thickness ( h ′) of the substrate. ( b ) Magnified optical image of arrays of μ-cells printed into a photocured layer of polyurethane (PU) doped with the luminophore DCM, (scale bar: 500 μm). Inset, cross-sectional s.e.m. image (coloured) showing substrate (green), DCM-PU (red), Si μ-cell (yellow), and air (blue), (scale bar: 25 μm). ( c ) Absorption and emission spectra of a DCM-PU thin film (thickness ~30 μm) on a glass substrate (thickness ~1 mm), with a DCM concentration of ~0.19 wt% (red: absorption of DCM-PU, green: absorption of PU, blue: emission of DCM-PU). ( d ) Picture of a completed module, before forming interconnects. The dashed box in the centre corresponds to the region shown in frame ( b ), the scale bar in this image is 2 mm. Full size image For the work presented here, bulk, p-type 〈111〉 Czochralski Si wafers (10–20 Ω·cm, Virginia Semiconductor Inc.) provide source materials for μ-cells formed by conventional processes of silicon microfabrication, including optical lithography, dry and wet-chemical etching and thermal diffusion for doping [18] . Techniques of transfer printing allow deterministic assembly of organized arrays of these μ-cells, in any spatial configuration. For experiments described here, plates of glass or sheets of polyethyleneterephthalate serve as substrates. Thin luminescent coatings, which we refer to as the LSC layers, consist of an ultraviolet-curable polyurethane (PU, Norland Products Inc.) matrix doped with an organic dye (DCM, (4-dicyanomethylene-2-methyl-6-p-dimethylaminostyryl-4H-pyran), Exciton). The printing process embeds the μ-cells at the near surface region of this layer, in a way that still allows unobstructed exposure of their top surfaces to incident light ( Fig. 1b ). The absorption and emission spectra of PU and DCM-doped PU (DCM-PU, ~0.19 wt%) in fully cured solid films appear in Figure 1c . The peak wavelengths for emission and absorption are 602 and 477 nm, respectively. The dye concentration is sufficiently high to provide strong absorption even for thin LSC layers, but sufficiently low to maintain high fluorescence yields ( Supplementary Information ). The backside reflector (BSR) consists of a black anodized aluminium plate, a silver mirror, or a white polyester cloth (TX609, Texwipe) mounted on the mirror, to provide non-reflective, specular and diffuse reflective conditions, respectively. The measured reflectivities for the specular, diffuse and non-reflective cases are 98, 93 and 22% averaged through the spectral range of 400–1,100 nm, respectively. Figure 1d shows a representative module consisting of sparse arrays of μ-cells printed directly into a DCM-PU LSC layer, on a glass substrate. 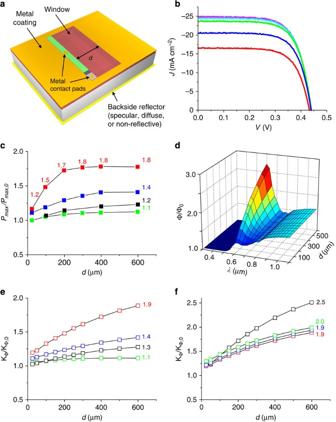Figure 2: Effect of illumination area and backside reflector on the performance of a top-mounted silicon solar μ-cell. (a) Schematic illustration of a single μ-cell in a layer of DCM-PU on a glass substrate with a lithographically defined metallic (Cr/Au: ~15 nm/400 nm) aperture (length: 1.6 mm, width:d). Three different BSRs were explored: specular and diffuse reflective, and non-reflective. Electrical contact pads (30 μm×50 μm) were formed by photolithography and evaporation of metals (Cr/Au: ~10 nm/150 nm). (b) Representative current density (J=current/top surface area of the μ-cell)—voltage (V) curves of a μ-cell under AM 1.5D illumination as a function of aperture width (d), with a specular BSR (d=23 (red), 96 (blue), 200 (green), 300 (cyan), 400 (pink), 600 (orange) μm). (c) Normalized maximum output power (Pmax/Pmax,0) of the μ-cell as a function ofd, with non-reflective (green), specular- (red) and diffuse-reflective (blue) BSRs. The case of a system without the DCM, with a diffuse-reflective BSR is also shown (black).Pmaxis the maximum output power due to the photon flux impinging through all surfaces of the cell, andPmax,0is the maximum output power due to the photon flux incident only through the top surface, as approximated by the maximum power evaluated atd=23 μm with a non-reflective BSR. (d) Contour plot of computed, normalized total photon flux density (Φ(d,λ)/Φ0(d,λ)) as a function of wavelength (λ) anddwith a specular BSR. Here Φ(d,λ) is the photon flux density absorbed through all surfaces of a μ-cell and Φ0(d,λ) is the flux density through only its top surface with a non-reflective BSR. (e) Integrated total photon flux (KΦ/KΦ,0) as a function ofd, with non-reflective (green), specular- (red) and diffuse-reflective (blue) BSRs, whereΦ is shown in (d). Corresponding data for the system without the DCM, with a diffuse-reflective BSR ,are also shown (black). (f) Integrated total photon flux (KΦ/KΦ,0) with specular reflective BSR, under various loss conditions where one of the loss mechanisms, including those associated with incomplete internal reflections (non-TIR; black), self-absorption (SA; blue) and imperfect BSR (green), is separately eliminated. A baseline (red) with all losses included is also shown. Study of a model luminescent solar concentrator with a single μ-cell To explore the optics, we first consider a simple model structure that consists of a single μ-cell ( t =15 μm, w =50 μm, h =24 μm, h ′=1 mm) implemented in an LSC system with variable illumination area, as illustrated in Figure 2a . The 15 μm thickness leads to ~54% absorption of light normally incident on the μ-cell in a double-pass configuration without anti-reflection (AR) coatings, averaged over the solar spectrum (300–1100nm), or ~75% in a single-pass configuration with a perfect AR coating on top surface. The 50 μm width enables higher levels of absorption (~85% for the case with a perfect AR coating) for light incident on the sides of the μ-cells, in a single pass. The 24 μm thick LSC layer absorbs ~92% of normally incident light at a wavelength of 477 nm in a double pass, or ~72% in a single pass. A metallic aperture (Cr/Au, ~15 nm/400 nm) allows incident light to expose only a certain area of the LSC immediately adjacent to the μ-cell. Electrical contact pads (30 μm×50 μm) formed by photolithography and electron beam evaporation (Cr/Au, ~10 nm/150 nm) exist at the end (p+) and middle (n+) of the μ-cell. Figure 2b shows the measured current density ( J = I / A 0 , where I is the current and A 0 is the top surface area of the cell) as a function of applied voltage ( V ), under simulated AM 1.5D illumination (1,000 W m −2 ) at room temperature, for several different aperture areas (1.6 mm× d μm, where d is the distance between the edges of the μ-cell and the aperture), with a specular reflective BSR. As d increases, the fill factor remains constant (~0.69) and the open circuit voltage ( V oc ) increases only slightly, while the short-circuit current density ( J sc ) increases significantly. These trends are all consistent with an increasing total photon flux into the μ-cell. Similar studies with non-reflective and diffuse reflective BSRs yield similar types of data. Results of normalized maximum output power ( P max / P max,0 ) extracted from such measurements appear in Figure 2c , where P max is the maximum total output power from the μ-cell, under conditions described above, and P max,0 is the maximum output power associated with photon flux incident only through the top surface of the μ-cell, as approximated by the maximum power evaluated at d =23 μm with a non-reflective BSR. In all cases, the performance monotonically increases with d , simply because additional photons are guided to the μ-cell. The rate of increase diminishes with d , due to propagation losses, geometric effects and others described subsequently. Measurements on a device with a diffuse BSR but without DCM (also in Fig. 2c ) show clearly that the μ-cell geometry allows effective capture of scattered photons incident on the bottom and sidewall surfaces, even without the LSC mechanism. For cases with DCM, P max / P max,0 asymptotically approach saturation values, P sat , at roughly d ~0.4 mm= d sat . This length scale is compatible with microscale, distributed solar cells, but not with conventional, bulk cells of previously reported LSC systems. Figure 2: Effect of illumination area and backside reflector on the performance of a top-mounted silicon solar μ-cell. ( a ) Schematic illustration of a single μ-cell in a layer of DCM-PU on a glass substrate with a lithographically defined metallic (Cr/Au: ~15 nm/400 nm) aperture (length: 1.6 mm, width: d ). Three different BSRs were explored: specular and diffuse reflective, and non-reflective. Electrical contact pads (30 μm×50 μm) were formed by photolithography and evaporation of metals (Cr/Au: ~10 nm/150 nm). ( b ) Representative current density ( J =current/top surface area of the μ-cell)—voltage ( V ) curves of a μ-cell under AM 1.5D illumination as a function of aperture width ( d ), with a specular BSR ( d =23 (red), 96 (blue), 200 (green), 300 (cyan), 400 (pink), 600 (orange) μm). ( c ) Normalized maximum output power ( P max / P max,0 ) of the μ-cell as a function of d , with non-reflective (green), specular- (red) and diffuse-reflective (blue) BSRs. The case of a system without the DCM, with a diffuse-reflective BSR is also shown (black). P max is the maximum output power due to the photon flux impinging through all surfaces of the cell, and P max,0 is the maximum output power due to the photon flux incident only through the top surface, as approximated by the maximum power evaluated at d =23 μm with a non-reflective BSR. ( d ) Contour plot of computed, normalized total photon flux density (Φ( d , λ )/Φ 0 ( d , λ )) as a function of wavelength (λ) and d with a specular BSR. Here Φ( d , λ ) is the photon flux density absorbed through all surfaces of a μ-cell and Φ 0 ( d , λ ) is the flux density through only its top surface with a non-reflective BSR. ( e ) Integrated total photon flux ( K Φ / K Φ,0 ) as a function of d , with non-reflective (green), specular- (red) and diffuse-reflective (blue) BSRs, where Φ is shown in ( d ). Corresponding data for the system without the DCM, with a diffuse-reflective BSR ,are also shown (black). ( f ) Integrated total photon flux (K Φ /K Φ,0 ) with specular reflective BSR, under various loss conditions where one of the loss mechanisms, including those associated with incomplete internal reflections (non-TIR; black), self-absorption (SA; blue) and imperfect BSR (green), is separately eliminated. A baseline (red) with all losses included is also shown. Full size image The data in Figure 2c provide some useful, qualitative insights. First, when d is close to zero, light capture arises mainly from direct illumination of the top surface of the μ-cell and from transmitted light that reflects from the BSR and enters back through the bottom surface. Consistent with the definitions described above, the non-reflective case has P max / P max,0 ~1. The device with diffuse BSR shows P max / P max,0 ~1.11. In this regime, the corresponding case without DCM exhibits similar behaviour, as expected due to the small thickness of the LSC material under the μ-cell. The specular case corresponds to full, double-pass operation. Here the value of P max / P max,0 ~1.17 is approximately consistent with the computed ratios of double-pass to single-pass absorption (without AR coating), that is, ~54%/~47%~1.15. This estimated value assumes d =0 μm, whereas the experiment uses d =23 μm. As d increases, P max / P max,0 improves for all device types, due to increases in photon capture via flux through the sidewalls and bottoms of the μ-cells, from scattered, reflected and waveguided photons, both luminescent and non-luminescent. The non-reflective device shows the smallest P sat , consistent with an overall concentration mechanism that relies largely on waveguided and reflected photons, most of which are eliminated by the non-reflective BSR. Compared with the case with DCM, the diffuse BSR device without DCM shows larger d sat , and smaller P max / P max,0 throughout the range of d shown here, due to the absence of absorption and emission associated with the DCM (the values of P sat for these two cases happen to be similar, due to a fortuitous balance of luminescence gains and collection losses, Supplementary Information ). The specular system shows higher P sat than an otherwise similar device with diffuse BSR, due primarily to favourable effects of the specular BSR on waveguiding. Numerical modelling supports these conclusions, and provides additional detail. Here results are presented for geometrical optics and a statistical Monte-Carlo technique that includes multiple scattering processes at various interfaces, as well as isotropic emission and self-absorption of the luminophores [19] , [20] . Photon transport in the LSC is considered via equations for spectral irradiance/radiance propagation in absorbing media with luminescent downconversion ( Supplementary Information ). The photon flux absorbed by a μ-cell is calculated as a summation over multiple propagation directions ( θ , φ ; see Fig. 1a ), with averaging over multiple azimuth angles, and multiple generations of rays, integrated over the whole spectrum: where F i ,abs ( λ , θ n , φ ) is the absorbed spectral irradiance, h is Planck's constant and c is the speed of light. Detailed information on this theoretical model will appear elsewhere. Figure 2d shows a contour plot of the normalized total photon flux density (Φ( d , λ )/Φ 0 ( d , λ )) as a function of wavelength ( λ ) and d with a specular-reflective BSR, where Φ( d , λ ) is the flux density absorbed through all surfaces of a μ-cell and Φ 0 ( d , λ ) is the flux density only through its top surface with a non-reflective BSR. Here, the strongest enhancements occur near wavelengths associated with emission from the DCM, as expected. The performance of the μ-cells depends on the integrated photon flux, K Φ ( d )/ K Φ,0 ( d ), where . This parameter can be compared directly with experimental values of P max / P max,0 , assuming that the output power increases linearly with absorbed photon flux. The results, presented in Figure 2e , show good agreement with experiment, without any fitting parameters. Discrepancies might arise from non-ideal waveguide geometries, surface roughnesses and other aspects of the experimental systems. These calculation techniques can be used to guide optimization and to evaluate the influence of different loss mechanisms, such as those due to incomplete internal reflections for photons that do not undergo TIR at the top surface (that is, non-TIR), absorption and non-radiative relaxation by the DCM for spectrally resonant photons (that is, self-absorption) and absorption at the BSR and other parasitic waveguide losses from scattering and related non-ideal features of the structures (that is, BSR and parasitic, respectively), both of which affect all photons. Modelling allows separate investigation of the effects of each of these loss mechanisms, except for parasitics, which are explicitly neglected. Figure 2f shows the calculated behaviour of the specular BSR case, when each mechanism is eliminated separately. Clearly, the non-TIR loss dominates. When the non-TIR mechanism is turned off, the K Φ ( d )/ K Φ,0 ( d ) at d =600 μm increases to ~2.5. Assuming a lossless BSR and no self-absorption results in only a slight improvement ( Fig. 2f ). Geometrical aspects associated with the thickness of the substrate, h ′, also affect the absorbed photon flux to the μ-cell. In particular, the solid angle subtended by a μ-cell from any point at the BSR surface decreases with increasing h ′. This effect influences the probability that a reflected photon is directed to the μ-cell. When h ′ is much larger than w , a large portion of the photon flux never interacts with the μ-cell. On the other hand, as h ′ decreases to zero, the effect of self-absorption and losses at the BSR can become significant due to confinement of light in the LSC layer. In particular, for LSC optical densities near unity, the propagation lengths due to re-absorption are comparable with the LSC thicknesses ( h ) that, by necessity, lie in the sub-mm range for flexible designs. These observations on behaviour for limiting cases of thick and thin substrates suggest that there exists an optimal value of h ′, where a few hundred microns provide a good balance. Performance of luminescent solar concentrator module with arrays of μ-cells On the basis of the understanding established by these experimental and modelling results, we considered module-level systems constructed using distributed arrays of μ-cells, with different spacings ( s ). 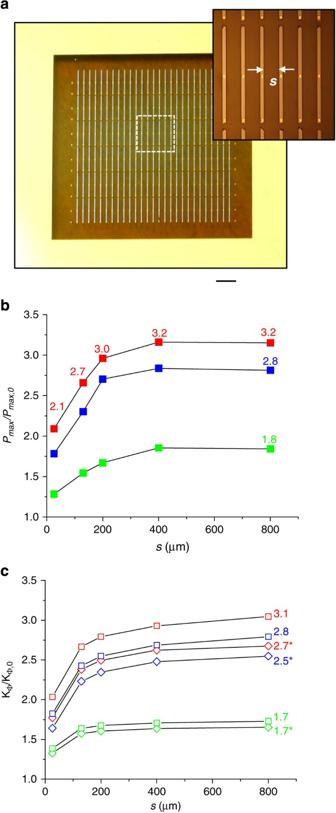Figure 3: Performance of an LSC system with arrays of silicon solar μ-cells. (a) Optical image of a system with cells in an array with a spacing (s) of 400 μm. The gold metallic aperture around the perimeter of the array restricts the total illumination area to 12.00 mm×11.83 mm (scale bar: 1 mm). Electrical contact pads (30 μm×50 μm) were formed by photolithography and evaporation of metals (Cr/Au: ~10 nm/150 nm). (b) Measured normalized maximum power (Pmax/Pmax,0) as a function ofs, measured on a μ-cell in the centre of the array, with non-reflective (green), specular- (red), or diffuse-reflective (blue) BSRs. (c) Calculated normalized total photon flux (KΦ/KΦ,0) for an individual, centrally located μ-cell as a function ofsunder non-reflective (green), specular- (red), or diffuse-reflective (blue) BSR conditions, with (square) and without (diamond, *) photon flux contributed from the perimeter of the array. Figure 3a shows a representative device, with s =400 μm. A metallic aperture (12.00×11.83 mm 2 ) lithographically defined around the perimeter of the each module ensures constant illumination area. Current-voltage characteristics evaluated on a single μ-cell near the centre of the array in each case provide metrics of module performance. A series of such measurements on modules, with a range of values of s , yield data qualitatively similar to those of Figure 2 (see Fig. 3b ). As observed in Figure 2 , the specular BSR shows better performance than diffuse or non-reflective BSRs, for similar reasons. The maximum improvement is ~320%, which corresponds to a situation where more than twice as many photons are indirectly collected through the sidewalls and bottom surfaces of the μ-cells than those directly incident on the top. The equivalent values of d sat for the array cases ( Fig. 3 ) are smaller than those for model systems ( Fig. 2 ), due to losses associated with the μ-cells in the former. Photon flux from both sides of the μ-cells in the arrays leads to values of ( P sat −1) that are expected to be, very roughly, two times greater than those for the model system. The illuminated areas, along the perimeter of the array, contribute additional photon flux to create somewhat larger differences; these contributions are most significant near s ~0, where the gaps between the μ-cells have a less significant role. Optical models described previously, but modified to accommodate the array layouts and the perimeter areas explicitly, yield values of ( K Φ ( s )/ K Φ,0 ( s )) ( Fig. 3c ) that exhibit good agreement with experimental data. Calculations without the perimeter areas, also shown in Figure 3c , show their effects. Figure 3: Performance of an LSC system with arrays of silicon solar μ-cells. ( a ) Optical image of a system with cells in an array with a spacing ( s ) of 400 μm. The gold metallic aperture around the perimeter of the array restricts the total illumination area to 12.00 mm×11.83 mm (scale bar: 1 mm). Electrical contact pads (30 μm×50 μm) were formed by photolithography and evaporation of metals (Cr/Au: ~10 nm/150 nm). ( b ) Measured normalized maximum power ( P max / P max,0 ) as a function of s , measured on a μ-cell in the centre of the array, with non-reflective (green), specular- (red), or diffuse-reflective (blue) BSRs. ( c ) Calculated normalized total photon flux (K Φ /K Φ,0 ) for an individual, centrally located μ-cell as a function of s under non-reflective (green), specular- (red), or diffuse-reflective (blue) BSR conditions, with (square) and without (diamond, *) photon flux contributed from the perimeter of the array. Full size image Mechanically flexible luminescent concentrator system PV systems with these configurations can accommodate a wide range of design choices, including challenging cases that require small thicknesses for mechanical bendability. To demonstrate this option, we built devices using the optimized designs ( s =400 μm, specular BSR) of Figure 3 on thin sheets of polyethyleneterephthalate (thickness ~50 μm), and in layouts that implement a top coating of PU (~30 μm) to yield a neutral mechanical plane layout [18] . The PU reduces the reflection losses at the surface of silicon, and also changes other optical characteristics of the structure. 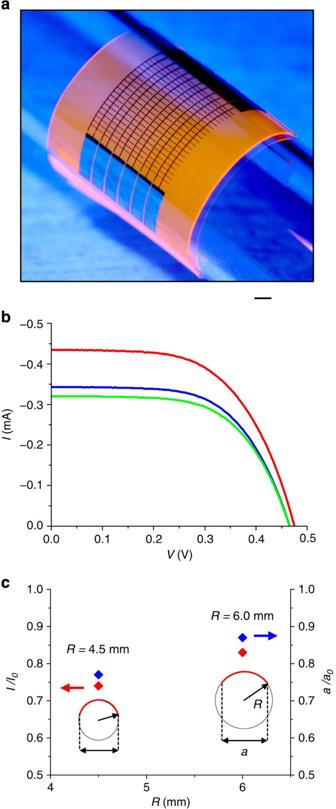Figure 4: Performance of a mechanically flexible luminescent solar module on a thin sheet of plastic. (a) Optical image of a representative device bent on a cylindrical support (scale bar: 1 mm). Each metal grid line interconnects 21 μ-cells, with cell-to-cell spacings of 400 μm. (b) Measured total output current (I) as a function of voltage (V) under AM 1.5D illumination, in flat (red) and bent states (bending radii of 6.0 mm (blue) and 4.5 mm (green)). (c) Ratio of measured short circuit currents (I/I0; red) and projected areas (a/a0; blue) between bent and flat states as a function of bending radius (R), whereI0(I) anda0(a) are the short circuit current and width of the module along the bending direction in the flat (bent) state, respectively. Figure 4a shows such a module bent on a cylindrical support. The array consists of 21 μ-cells interconnected with metal grid lines. The total current produced under AM 1.5D illumination, in flat and bent states (two different radii of curvature, R ), appears in Figure 4b . Owing to several differences in design, quantitative comparison against the modules of Figure 3 is not straightforward. The current densities per cell are, however, comparable: ~41 mA cm −2 for the specular BSR system ( s =400 μm) of Figure 3 , and ~31 mA cm −2 for the case of Figure 4 , the latter of which includes Ohmic losses and other adverse effects, including μ-cell variability, that reduce the performance. The output power decreases when bent, mainly due to the decrease in flux associated with reductions in projected area normal to the incident light rather than any fundamental change in the efficiency of the concentration. The short circuit currents measured in these bent states decrease to ~83% ( R =6.0 mm) and ~74% ( R =4.5 mm) of values in the flat state. The corresponding reductions in the projected areas are 87 and 77% ( Fig. 4c ), thereby providing an explanation for the observed behaviour. Reflection losses associated with oblique illumination are negligible ( Supplementary Information ). Numerical modelling suggests that bending can increase the fraction of incident photons that are coupled into the collector in the wavelength range that luminophores do not absorb, to provide additional indirect flux into the μ-cells. Additionally, photons incident on the system at oblique angles have increased path lengths through the LSC, contributing to slightly more efficient luminescent conversion. Detailed theoretical studies of these and related effects will appear in a separate publication. Figure 4: Performance of a mechanically flexible luminescent solar module on a thin sheet of plastic. ( a ) Optical image of a representative device bent on a cylindrical support (scale bar: 1 mm). Each metal grid line interconnects 21 μ-cells, with cell-to-cell spacings of 400 μm. ( b ) Measured total output current ( I ) as a function of voltage ( V ) under AM 1.5D illumination, in flat (red) and bent states (bending radii of 6.0 mm (blue) and 4.5 mm (green)). ( c ) Ratio of measured short circuit currents ( I / I 0 ; red) and projected areas ( a / a 0 ; blue) between bent and flat states as a function of bending radius ( R ), where I 0 ( I ) and a 0 ( a ) are the short circuit current and width of the module along the bending direction in the flat (bent) state, respectively. Full size image The collection efficiency of this type of LSC system can be defined by considering the output power, the total illumination area ( A ) of the collector and the summed area of the μ-cells ( n × A 0 , where n is the number of μ-cells). For simplicity, consider the case of Figure 2a , where n =1 and we can write: Here, I 0 is the intensity of incident solar radiation, η col is the optical efficiency of the LSC system, and η cell is power-conversion efficiency of a μ-cell. At d =200 μm, A =4· A 0 and P max =1.7· I 0 · A 0 · η cell . The collector efficiency is therefore 0.7/4 ~17.5%. The corresponding efficiency for the system without DCM using diffuse BSR is 0.14/4 ~3.5%. The same definition can be applied to the module of Figure 3 . To minimize edge effects, we consider the collector efficiency only for regions near the centr. Here, at s =400 μm the efficiency is approximately 2.2/8 ~27.5% ( P max =3.2· I 0 · A 0 · η cell , A =8 A 0 ). By similar metrics, conventional LSC systems offer collection efficiencies in the range of 4–7% [21] . As shown clearly in Figures 2 and 3 , the output power saturates with increasing d ; this behaviour leads to a decrease in η col at large d . For example, η col ~0.8/8=10% for d =400 μm; the efficiency is negligible in the limit of large d . The total power conversion efficiency is less than that of an otherwise similar module but with full area coverage of silicon microcells. The power produced by the LSC system is, however, 320% larger than that possible with the same microcells but without concentration. The unusual LSC designs reported here offer improved performance compared with conventional layouts, and a variety of engineering options with particular value in ultrathin, lightweight and bendable systems. For practical applications that require stability under long-term exposure to sunlight, inorganic quantum dot luminophores might provide attractive alternatives to the organic dyes used here. The computational models and underlying concepts are compatible with other more advanced luminophores (for example, quantum dots), solar cells (for example, compound semiconductor devices) and waveguide structures (for example, photonic crystals). Multilayer systems with additional optical elements and structures for spectral splitting can also be envisioned. The rich range of design and materials possibilities suggests multiple paths for optimization. Fabrication and measurement Monocrystalline silicon μ-cells were fabricated from p-type 〈111〉 Czochralski Si wafers (10–20 Ω·cm, Virginia Semiconductor Inc.) as reported previously [18] . The resulting devices were printed individually or as arrays on glass or polyethyleneterephthalate substrates coated with a thin (~30 μm) luminophore-containing polymer layer. For the single μ-cell experiments, a metallic aperture was defined by electron-beam evaporation (Cr/Au; 15 nm/400 nm), photolithography and wet chemical etching. Electrical contact pads (30 μm×50 μm) at the end (p+) and middle (n+) of the μ-cell were formed by photolithography and evaporation of metals (Cr/Au: ~10 nm/150 nm). The luminescent medium consisted of an ultraviolet-curable polyurethane (NOA61, Norland Products Inc.) mixed with an organic laser dye (DCM, Exciton). The mixing used methyl ethyl ketone as a co-solvent followed by vacuum removal of the solvent. Absorption and emission spectra of fully cured layers (thickness ~30 μm) of PU and DCM-PU (~0.19 wt%) on glass substrates were measured using a CARY 5G spectrophotometer. Black anodized aluminium (Al) plates, Ag-coated metallic mirrors and white polyester cloth (TX609, Texwipe) attached on such mirrors provided non-reflective, specular- and diffuse-reflective BSRs, respectively. The reflectivity of the BSR was measured using a Cary 5G spectrophotometer with a diffuse reflectivity accessory, where teflon powder standard (Spectralon, Labsphere) was used as 100% reflectivity reference. The PV characteristics of the μ-cells and modules were measured using a source meter (model 2400, Keithley) and a 1,000 W full spectrum solar simulator (Oriel, 91192). Bending experiments were conducted with modules attached to glass test tubes (VWR) with outer surface diameters of 12 and 9 mm. Numerical calculation A ray-tracing model was implemented as a Matlab code, with a grid resolution of 5 μm for the BSR, PU-air and semiconductor-PU, and semiconductor-air surfaces. The distances travelled along the ray paths between two luminescent emission events were 5 μm. The difference between the integrated photon fluxes, calculated with 2 and 10 μm resolutions, was less than 0.5%, thus justifying the spatial discretization of 5 μm. The stochastic error in the absorbed photon flux for the 120,000 rays used in simulations is expected to be <0.3% of the mean value for the 5 μm discretization. The total number of rays considered in each of 6 generations was 120,000 (sampling 600 elevation angles between [−π/2, π/2] and 200 azimuth angles between [−π, π]). Both ray elevation and azimuth angles had uniform random distributions. The μ-cells were considered to extend infinitely along the third dimension. In this sense, the model is two-dimensional, but it used reflection coefficients and ray path lengths averaged over multiple azimuth directions to account for the third dimension (that is, along the lengths of the μ-cells). The propagating photon fluxes at the edges of the structure were terminated with absorbing boundary conditions. The angular spectrum of the diffuse reflector was assumed to be Lambertian. Fresnel reflection, and transmission coefficients were calculated as the average of the values for transverse magnetic and transverse electric polarizations, thus, assuming random polarization of incident light. All the spectral material properties as well as solar spectrum itself were interpolated at 60 uniformly spaced discrete wavelengths from 300 to 1,100 nm. The luminescent dye was assumed to have the quantum yield of 0.99. We note that the two-dimensional (2D) approximation associated with the procedures described above ignores light that escapes beyond the edges of the μ-cell, in the setup of Figure 2 . For all calculations pertaining to Figure 2 , we used a scaling function that accounts for the finite aperture, based on geometrical optics solution. A numerical solution of an equivalent three-dimensional (3D) radiative transfer problem in the diffusion approximation suggests a reduction of ~11% in the photon flux absorbed in the μ-cell for the 3D case compared with 2D at d =400 μm. The geometrical optics model suggests ~17% reduction for the same case. How to cite this article: Yoon, J. et al . Flexible concentrator photovoltaics based on microscale silicon solar cells embedded in luminescent waveguides. Nat. Commun. 2:343 doi: 10.1038/ncomms1318 (2011).